Casimir–Polder interactions in the presence of thermally excited surface modes The temperature dependence of the Casimir–Polder interaction addresses fundamental issues for understanding vacuum and thermal fluctuations. It is highly sensitive to surface waves, which, in the near field, govern the thermal emission of a hot surface. Here we use optical reflection spectroscopy to monitor the atom–surface interaction potential between a Cs*(7D 3/2 ) atom and a hot sapphire surface at distances of ~100 nm. In our experiments, that explore a large range of temperatures (500–1,000 K), the surface is at thermal equilibrium with the vacuum. The observed increase of the interaction with temperature, by up to 50%, relies on the coupling between atomic virtual transitions in the infrared range and thermally excited surface-polariton modes. We extrapolate our findings to a broad distance range, from the isolated atom to the short distances relevant to physical chemistry. Our work also opens the prospect of controlling atom–surface interactions by engineering thermal fields. At the onset of the twentieth century, the spectral behaviour of black-body radiation (BBR), although a prototype of an incoherent source, has inspired the quantization of the electromagnetic field. It also inevitably led to the recognition of the existence of zero-point energy, the so-called vacuum fluctuations. Vacuum fluctuations are ultimately responsible for the finite lifetime (spontaneous emission) and a displacement of the energy states of an isolated atom (Lamb shift). In a ‘hot’ vacuum (vacuum and thermal fluctuations), both lifetime and Lamb shift exhibit a temperature dependence [1] , [2] whose influence becomes increasingly important for ultimate optical clocks [3] . Vacuum fluctuations are also responsible for the Casimir force, an attraction between two neutral bodies such as two metallic surfaces, currently considered to be of utmost fundamental importance, while also playing a considerable role in Micro and Nano-Electro-Mechanical Systems [4] . For Casimir effect studies, an exact evaluation of the temperature corrections is still required for a comparison between theory and high-precision experiments [5] , [6] , [7] , [8] , which until now have always been performed at room temperature [9] , [10] . Closely related is the long-range atom–surface interaction, now generically described as the Casimir–Polder (CP) effect [11] , [12] . It is of practical relevance for devices that trap atoms or molecules close to a surface, such as chips or nanofibres, intended for quantum information processing experiments [13] , [14] . Again, temperature corrections may play a key role, as exemplified by measurements embarked on the search of exotic non-Newtonian gravity force [15] . Until now, the only measurement demonstrating a temperature dependence of the CP attraction was performed at distances 7–11 μm, where the interaction is extremely small [16] . Critical to experimental success was an enhancement due to an out-of-equilibrium effect [17] , where the surface is held at a higher temperature than the surrounding vacuum. In the near-field regime, thermal emission exhibits properties radically different from those of the (far-field) BBR [18] , including spatial coherence [19] and a spectrum intimately related to the resonances of the material through surface modes [20] . For distances smaller than 100 nm, the CP interaction is in the van der Waals (vW) regime [11] , which resembles the interaction between a fluctuating dipole and its electrostatic image in front of the surface. It is characterized by a – C 3 . z −3 potential, where z is the atom–surface distance and C 3 is the vW coefficient [21] . In contrast to the far-field regime analysed in refs 16 , 17 , the near-field CP interaction strongly depends on the dielectric properties of the surface, especially when surface modes coincide with atomic resonances [22] . The coupling between atoms (in the vacuum side) and surface polaritons can lead to exotic effects such as atom–surface giant attraction ( C 3 >0), or even repulsion ( C 3 <0). A negative C 3 was experimentally demonstrated in the past [23] , [24] for Cs*(6D 3/2 ) against a sapphire surface. Further extension to a Förster-like real energy transfer of the atomic excitation into a surface mode was also observed [25] . This resonant atom–surface enhanced process was intrinsically restricted to excited atoms at zero temperature ( T =0). Conversely, when surface polariton modes are thermally populated [23] , [26] , [27] , the atom surface coupling is not limited to an atomic virtual emission, but can be reversed, and the vicinity with the surface can induce a virtual or real atomic excitation. With respect to the mean occupation number of photons of energy ħω , , only low-energy atomic transitions should contribute to this type of thermal effects: at room temperature, only modes of wavelength >50 μm are significantly populated. This suggests that only excited high-lying state atoms or even molecules could be sensitive to temperature effects in the near-field regime, while ground state atoms are typically excluded. Here we report on spectroscopic measurements of the vW coefficient between a Cs*(7D 3/2 ) atom and a sapphire surface as a function of temperature. We briefly discuss the theoretical predictions that justify the particular choice of the atom–surface system and present experimental observations of a sensitive temperature dependence of the CP interaction at distances on the order of 100 nm. We extrapolate our findings to a broad distance range and discuss applications that could stem from our work. Before discussing our experimental findings, we first describe the theoretical reasoning behind the choice of the specific atom–surface system. The vW coefficient for a given | i › level sums up the contributions of all allowed dipole couplings | i ›→| j › of frequency ω ij , considered negative in the case of virtual emission. For our experiment a schematic diagram of the Cs energy levels and the relevant couplings is shown in Fig. 1a . For an ideal conductor, one obtains simply , with ‹ i | D | j › the dipole moment matrix elements. 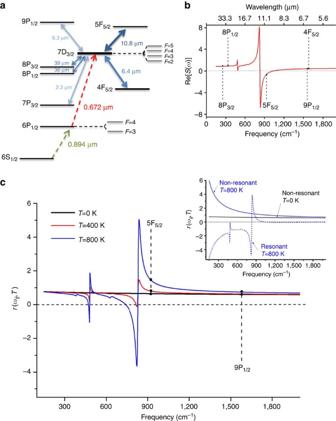Figure 1:Atom–surface system. (a) The Cs energy levels and the dipole transitions relevant to our experiment. The dashed arrows represent the optical excitation scheme, with pumping from the ground 6S1/2and probing from the 6P1/2level. (b) The real part of the sapphire surface response, Re[S(ω)]. We use experimental measurements performed at room temperature given in ref.39. The solid points show the positions of the relevant dipole coupling from 7D3/2. (c) The image coefficient of a sapphire surface for a virtual atomic absorption (ωij>0) as a function of the transition frequency forT=0 K,T=400 K andT=800 K. The inset shows separate plots of resonant (dashed) and non-resonant (solid) contributions forT=800 K and forT=0 (resonant term is zero). One notes that the monotone behaviour predicted atT=0 disappears at finite temperatures. In the case of a real dielectric, each contribution is individually weighed by an image coefficient r ( ω ij , T ), given below [27] : Figure 1: Atom–surface system . ( a ) The Cs energy levels and the dipole transitions relevant to our experiment. The dashed arrows represent the optical excitation scheme, with pumping from the ground 6S 1/2 and probing from the 6P 1/2 level. ( b ) The real part of the sapphire surface response, Re[ S ( ω )]. We use experimental measurements performed at room temperature given in ref. 39 . The solid points show the positions of the relevant dipole coupling from 7D 3/2 . ( c ) The image coefficient of a sapphire surface for a virtual atomic absorption ( ω ij >0) as a function of the transition frequency for T =0 K, T =400 K and T =800 K. The inset shows separate plots of resonant (dashed) and non-resonant (solid) contributions for T =800 K and for T =0 (resonant term is zero). One notes that the monotone behaviour predicted at T =0 disappears at finite temperatures. Full size image In equation (1), the first term, sometimes called ‘non-resonant’, resembles a distance-dependent Lamb shift due to vacuum and thermal fluctuations covering the entire frequency spectrum. Here, u is the integration variable, S ( ω )=[ ε ( ω )−1]/[ ε ( ω )+1] is the surface response (see Fig. 1b for sapphire), with ε ( ω ) the complex bulk permittivity of the window, and f (ω ij , T , u ) is a generic function that groups all other contributions and turns the integral into a discreet sum over the Matsubara frequencies, when T ≠0. The second term, often called ‘resonant’, is reminiscent of the interaction between a classical oscillating dipole and its own reflected field [28] , [29] . For virtual absorption ( ω ij >0), it is simply proportional to the surface response at the atomic frequency and the mean photon occupation number n ( ω ij >0, T ), hence null at T =0 (ref. 22 ). For a virtual emission ( ω ij <0) the sign is inverted and one has to account for one additional photon due to spontaneous emission, so that . In Fig. 1c , we show the image coefficient of sapphire for a virtual absorption at different temperatures. A large temperature dependence is observed for virtual transitions whose frequency is in the vicinity of the surface polariton at 12.1 μm (830 cm −1 ). For smaller frequencies, the two terms of equation (1) tend to compensate (inset of Fig. 1c ) and temperature effects are smaller. This compensation is perfect only in the case of a dispersion-less ideal conductor [30] . Interestingly, in the high-frequency side of the spectrum, a small but non-negligible temperature dependence is observed, despite the small number of average photons present. This can be traced back to sapphire dispersion as well [31] . In the case of virtual emission, the temperature dependence of the image coefficient is analogous and adds to the resonant behaviour at T =0 mentioned above. Table 1 shows the contributions of each dipole coupling relevant for Cs*(7D 3/2 ). Remarkably, the 7D 3/2 →5F 5/2 virtual absorption at 10.8 μm, responsible for only half of the C 3 value at low temperature, carries nearly all of the C 3 temperature dependence. Conversely, the two important virtual atomic emissions 7D 3/2 →8P 1/2 at 29 μm and 7D 3/2 →8P 3/2 at 39 μm, exhibit only small temperature dependence despite their small energy. Table 1 Contributions of individual atomic transitions. Full size table For our experimental demonstration, we use selective reflection (SR) spectroscopy on the 6P 1/2 → 7D 3/2 line ( λ =672 nm), with a prior pumping step 6S 1/2 → 6P 1/2 ( λ p =894 nm). Linear SR spectroscopy on the interface between a dielectric and an atomic vapour is a long established spectroscopic method, in which the changes of the reflectivity coefficient near the atomic resonance yield information on the vapour spectrum close to the surface, typically probing a λ /2 π depth (~100 nm) largely compatible with the vW regime. SR spectroscopy, in its frequency-modulated version, has been rendered suitable for an accurate evaluation of the vW distance-dependent transition shift through numerous successive developments [21] , [23] , [24] , [32] , [33] , [34] , [35] . Here we use an intense beam at 894 nm, resonant with the 6S 1/2 → 6P 1/2 transition, which creates an almost uniform population of Cs*(6P 1/2 ) atoms. SR spectroscopy is then performed on the 6P 1/2 → 7D 3/2 line with a weak probe beam at 672 nm. Our experimental set-up ( Fig. 2a ) is similar to the one previously described in refs 23 , 24 . Our experiment essentially measures the temperature dependence of the interaction between sapphire and Cs*(7D 3/2 ), as the attraction exerted on Cs*(6P 1/2 ) is negligible (<2 kHz μm 3 ) [35] . 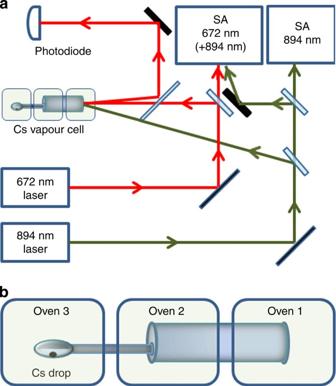Figure 2: Experimental set-up and Cs vapour cell. (a) Schematic of the experimental set-up. The essential experiment is a frequency-modulated (FM) SR at normal incidence at 672 nm, the oblique irradiation at 894 nm beam pumps the atoms to the intermediate 6P1/2level; the two SA experiments, at 894 nm (6S1/2→6P1/2), and at 672 nm (6P1/2→7D3/2), are respectively used for the locking and monitoring of the laser frequencies. (b) Schematic of the heated Cs cell with sapphire windows showing the differential heating, allowing separate control of the atomic vapour density, and of the window temperature. Figure 2: Experimental set-up and Cs vapour cell. ( a ) Schematic of the experimental set-up. The essential experiment is a frequency-modulated (FM) SR at normal incidence at 672 nm, the oblique irradiation at 894 nm beam pumps the atoms to the intermediate 6P 1/2 level; the two SA experiments, at 894 nm (6S 1/2 →6P 1/2 ), and at 672 nm (6P 1/2 →7D 3/2 ), are respectively used for the locking and monitoring of the laser frequencies. ( b ) Schematic of the heated Cs cell with sapphire windows showing the differential heating, allowing separate control of the atomic vapour density, and of the window temperature. Full size image Our measurements are conducted in an all-sapphire Cs vapour cell, shown in Fig. 2b . Sapphire has the benefit of being a robust material, reliable enough to allow the construction of a high-temperature cell [36] that operates at temperatures exceeding 1,000 K. The window, on which the SR experiment is performed, is ‘super-polished’ and post annealed with an average roughness of~0.3 nm, measured by atomic force microscopy. A differential heating system allows an independent control of the Cs vapour density, which is governed by a low-temperature reservoir usually operated in the range of ~400–450 K. A separate oven controls the temperature of the window, which is in equilibrium with its surrounding environment. This temperature T , varied between 500 and 1,000 K, is the one relevant for the atom-surface interaction. Experimentally, we scan the frequency of the 672-nm laser, sent under a near-normal incidence on the hot sapphire window, around one of the ensemble of resolved hyperfine components, that is, either the 6P 1/2 ( F =4) → 7D 3/2 { F ′=3,4,5}, or the 6P 1/2 ( F =3) → 7D 3/2 { F ′=2,3,4} transitions (see Fig. 1a ). An auxiliary saturated absorption (SA) experiment is implemented ( Fig. 2a ) to provide frequency markers of the free-atom spectrum. As in refs 23 , 24 , 33 , 34 , 35 , and thanks to the linearity of SR spectroscopy, a universal theoretical model [32] , taking into account the spatially inhomogeneous vW shift of the transition, the transient regime of optical interaction for moving atoms and the atomic velocity distribution, is used to fit the recorded spectra. The adjustable parameters are the vW coefficient ( C 3 ) and the linewidth of the atomic transition ( Γ ). In Fig. 3a , we present experimental spectra measured at the lowest ( T =490 K) and the highest ( T =1,000 K) window temperature. One notes the tremendous influence of the atom–surface interaction (see inset for C 3 =0) and important differences in the spectra when changing temperature. The theoretical fits are in very good agreement and the difference with the experimental curves is hardly visible at this scale. The linewidth of the atomic transition is kept constant in both experiments so that the changes in the shape of the spectra can be traced directly back to the change of the C 3 coefficient. 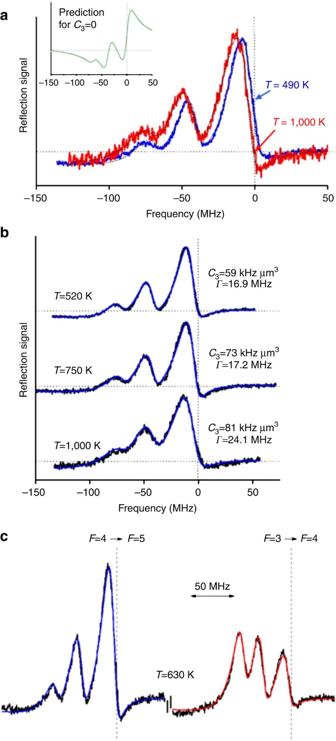Figure 3: Experimental spectra and theoretical fits. (a) Normalised frequency modulated (FM) SR spectra on the 6P1/2(F=4) → 7D3/2(F'=3, 4, 5) transition (672 nm) for a window temperature atT=490 K (blue) and atT=1,000 K (red). The frequency axis is referenced to the hyperfine component of the 6P1/2(F=4) →7D3/2(F'=5) transition as determined by the auxiliary SA. In the inset, we show the predicted FM SR spectrum in the absence of atom–surface interaction, that is,C3=0. The observed shift and lineshape distortion of the experimental curves are a clear evidence of the atom–surface interaction. The lower signal/noise ratio for 1,000 K window is further discussed in the Methods section. The dashed black lines are the respective theoretical fits, demonstrating the same linewidth for both temperaturesΓ=19 MHz and an increase ofC3with temperature from 55 to 86 kHz μm3(b) Experimental spectra (black) for FM SR at theF=4 →F'={3,4,5} hyperfine manifold for various window temperatures along with the corresponding theoretical fits (blue). The parameters used to fit the spectra are also indicated. (c) Experimental measurements (black) with their respective theoretical fits forF=4 →F'={3,4,5} (blue) andF=3 →F'={2,3,4} (red) manifold at identical conditions for both window temperature and vapour pressure/density. Despite the difference in the shape of the curves, the fit gives identical values for bothC3=64 kHz μm3andΓ=16 MHz. The window temperature isT=630 K. Figure 3b presents several other spectra for three indicative values of the window temperature ( T =520 K, T =750 K and T =1,000 K). Excellent fittings are observed in all cases and the evolution of the fitting parameters demonstrates a clear increase of the strength of the atom–surface interaction with temperature. We have performed various independent tests to check the consistency of our measurements, in the same way as in ref. 23 . For a given window temperature, we notably vary the Cs vapour pressure by changing the reservoir temperature, therefore changing the value of Γ due to collision broadening. These changes, although affecting the amplitude and shape of our spectra, do not modify the fitted C 3 values. In addition, when comparing the two different hyperfine manifolds, one observes strong differences in the overall shape of the curves owing to the different relative weight of each hyperfine transition, but identical values for C 3 and Γ are extracted for both spectra ( Fig. 3c ). Our measurements were also performed for many different spots on the sapphire window, with no significant changes. This is a crucial point because local structure variations (for example, roughness) or impurities (defects or ions) may severely affect atom–surface interaction and bias our measurements [37] , [38] . Consistent measurements were even found for a set of preliminary measurements performed in a sapphire cell with a lower surface quality. These precautions also assure us that no chemical degradation of the surface occurs with continuous exposure on chemically aggressive alkali vapour at elevated temperatures. Previous efforts to look for strong thermal effects predicted to occur at moderate temperatures for Cs*(8P) [34] , [35] , [39] close to fluoride windows whose surface resonances fall in the 30–40 μm range had turned out to be unsuccessful [40] due to the extreme mechanical and thermal fragility of fluoride windows. On the contrary, sapphire has been remarkably stable under these extreme conditions. Figure 3: Experimental spectra and theoretical fits. ( a ) Normalised frequency modulated (FM) SR spectra on the 6P 1/2 ( F =4) → 7D 3/2 ( F '=3, 4, 5) transition (672 nm) for a window temperature at T =490 K (blue) and at T =1,000 K (red). The frequency axis is referenced to the hyperfine component of the 6P 1/2 ( F =4) →7D 3/2 ( F '=5) transition as determined by the auxiliary SA. In the inset, we show the predicted FM SR spectrum in the absence of atom–surface interaction, that is, C 3 =0. The observed shift and lineshape distortion of the experimental curves are a clear evidence of the atom–surface interaction. The lower signal/noise ratio for 1,000 K window is further discussed in the Methods section. The dashed black lines are the respective theoretical fits, demonstrating the same linewidth for both temperatures Γ =19 MHz and an increase of C 3 with temperature from 55 to 86 kHz μm 3 ( b ) Experimental spectra (black) for FM SR at the F =4 → F '={3,4,5} hyperfine manifold for various window temperatures along with the corresponding theoretical fits (blue). The parameters used to fit the spectra are also indicated. ( c ) Experimental measurements (black) with their respective theoretical fits for F =4 → F '={3,4,5} (blue) and F =3 → F '={2,3,4} (red) manifold at identical conditions for both window temperature and vapour pressure/density. Despite the difference in the shape of the curves, the fit gives identical values for both C 3 =64 kHz μm 3 and Γ =16 MHz. The window temperature is T =630 K. Full size image Our experimental results are summarized in Fig. 4 . The experimental error bar for C 3 is on the order of 15% when fitting a single spectrum (see Fig. 7 of ref. 40 ), but reduces down to 5–10% after using all our independent measurements. One observes a significant increase of the vW coefficient with temperature (~50% from 500 to 1,000 K), which is in excellent agreement with the theoretical prediction, unambiguously demonstrating the fundamental thermal effects on the CP interaction. Our prediction requires the knowledge of the transition probabilities [41] and of the dielectric constant of sapphire on the entire spectrum. This introduces some small uncertainty in the theoretical values. The major contributing factor comes from the transition probabilities, which are not accurately known for all dipole couplings. We use theoretical estimates given in ref. 41 to which we moderately assign a 5% uncertainty. In Fig. 4 , we also show theoretical predictions using two different sets of experimental measurements [39] , [42] of the sapphire dielectric constant. The former [39] analyses in detail the effects of temperature (up to 800 K) on the dielectric constant of sapphire. The latter [42] also provides data for the sapphire dielectric constant on the extraordinary axis, which, in our experiment, is perpendicular to the window. Taking sapphire birefringence into account [43] has a small effect on our theoretical predictions. Further calculations show that the atom–surface interaction is independent of the actual axis orientation of sapphire to within 1%. Note that the uncertainties of the dielectric constant of sapphire may have a significant impact if a virtual transition coincides with surface polariton frequency. 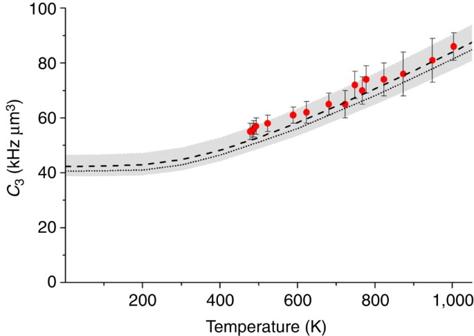Figure 4: Experiment versus theory. TheC3(van der Waals) coefficient as a function of temperature: red points represent experimental measurements. The dotted and dashed lines, respectively, represent theoretical predictions using the dielectric constant of sapphire reported in refs39,42. The grey shaded area of 5% plotted around the theoretical curves represents the uncertainty assigned to the transition probabilities. Figure 4: Experiment versus theory. The C 3 (van der Waals) coefficient as a function of temperature: red points represent experimental measurements. The dotted and dashed lines, respectively, represent theoretical predictions using the dielectric constant of sapphire reported in refs 39 , 42 . The grey shaded area of 5% plotted around the theoretical curves represents the uncertainty assigned to the transition probabilities. Full size image To extrapolate our findings to a larger scope and a variety of regimes, we also considered the effects of propagation for our Cs*(7D 3/2 )/sapphire system. 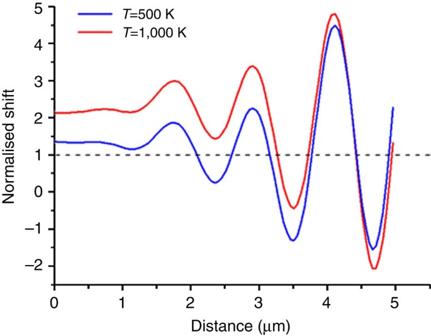Figure 5: Distance dependence of the CP interaction. Spatial dependence of the free energy shift of the Cs(7D3/2) atom in front of a sapphire surface, forT=500 K (blue) and 1,000 K (red), normalized to the spatially varying van der Waals electrostatic limit, −C3(T=0)/z3(dashed black line). Figure 5 shows for various temperatures the spatial evolution of the atom–surface interaction potential, as determined through a full quantum electrodynamics calculation. It confirms the validity of the – C 3 z −3 vW limit at any temperature for distances up to 100–200 nm, typically probed by SR spectroscopy. The typical evolution of the shift of a ground state atom, from z −3 (vW) to z −4 (CP asymptotic limit), and then after distances greater than the ‘thermal length’ back to z −3 (Lifshitz regime) [16] , [17] , is unnoticeable. Rather, the major correction to the vW limit is an oscillating behaviour from attraction to repulsion with an envelope decreasing slower than z −3 , typical of an excited atom due to the reflection of spontaneous emission [28] . In particular, the major contribution to oscillations comes from the 7D 3/2 →7 P 3/2 transition at 2.33 μm for which propagation effects ‘switch on’ much closer to the surface. Temperature dependence is small in this distance regime due to the absence of thermal photons at this wavelength. Thermal effects are the strongest in the near field as a consequence of the surface polariton. We point out here that our calculations give the free energy shift (see ref. 27 and references therein) due to the presence of the hot surface, ignoring the effects of BBR on an isolated atom. Taking into account this effect, discussed in detail in ref. 1 , the thermal contribution to the CP shift is dominant only when the atom is <1 μm away from the surface. Figure 5: Distance dependence of the CP interaction. Spatial dependence of the free energy shift of the Cs(7D 3/2 ) atom in front of a sapphire surface, for T =500 K (blue) and 1,000 K (red), normalized to the spatially varying van der Waals electrostatic limit, − C 3 ( T =0)/ z 3 (dashed black line). Full size image The distance limit that our experiments explore extends down to the nanometric range (~1 nm). This distance is already in the asymptotic ‘long-distance’ limit for various physical chemistry processes, of interest for a priori calculations [44] , [45] . Our result demonstrating that the CP attraction increases with temperature contradicts the generally accepted behaviour of thermal desorption. This should, nonetheless, be taken with a grain of salt, as the vW potential measured here is for an atomic excited state. However, our fundamental studies can provide new insights for the microscopic understanding of physico-chemical processes. As an example, in a temperature-dependent desorption process the thermally excited surface modes may selectively enhance a channel of energy transfer [46] , thus favouring a particular energy state for the desorbed atom or molecule. In conclusion, we have established that the interaction between a Cs*(7D 3/2 ) atom close to a hot sapphire surface, in thermal equilibrium with the environment, increases with temperature. This effect relies on the coupling of atomic excitations to surface polariton modes, which is critical in the vW regime of distances. A very good quantitative agreement with theory is observed. The influence of temperature reveals the quantum electrodynamics nature of the van der Waals interaction and may provide a useful knob to control forces between neutral atoms and surfaces up to their complete cancellation or change of sign. It is in particular possible to extend, with temperature as an extra parameter, the current studies on the Casimir interaction with specially designed nano- or microstructured surfaces, where the shaping allows tailoring the thermal field and possibly the interaction (repulsion and torque). Atoms may also be used as sensitive quantum probes of coherent thermal fields [19] or even of the correlated properties of thermal emission [47] , [48] . An alternative geometry would be a thin vapour cell [38] , [49] , which is a simple realization of a dielectric cavity, and an example of a situation where the temperature-dependence of surface interaction should depend on the surface geometry [50] . Thermal equilibrium in the vapour cell A schematic of the specially designed Cs cell, prepared by the group of D. Sarkisyan (Ashtarak, Armenia), is shown in Fig. 2b . It consists of a 10-cm-long cylindrical sapphire tube onto which two sapphire windows are glued. The primary window is ‘super-polished’ with the c axis perpendicular to the surface. It has a small wedge allowing us to select the reflection from the vapour interface. The mineral gluing is capable to resist temperatures up to 1,200 K. The secondary window is of a lower surface quality. The 7-cm-long sidearm, parallel to the cell’s main body, is glued on a small hole drilled on the secondary window. For this sidearm Cs cell, we have implemented a multiple section oven around the whole cell. Oven 1, ~5 cm long, controls the temperature of primary window region. It keeps the sapphire window in thermal equilibrium with the surrounding BBR. The temperature inside oven 1 can be chosen in the 500–1,000 K range. For such temperatures, the Cs vapour pressure would be considerable, and pressure broadening too high for any meaningful SR measurements. Ovens 2 and 3, also ~5 cm long each, impose a large temperature gradient on the entire cell and keep the sidearm as a ‘cold spot’ of the cell, where Cs condenses in liquid form. Oven 3 controls the temperature of the sidearm and, therefore, the Cs vapour pressure inside the cell. It is typically kept at temperatures around 400–450 K corresponding to a Cs equilibrium atom density ~10 14 –10 15 cm −3 . The temperature of each oven is measured with thermocouples, whose location can be moved, to evaluate the temperature homogeneity of the oven. Our readings inside oven 1 confirm that temperature is homogeneous to within 10–20 K. It is important to notice that the implementation of the differential heating in the Cs cell generates a temperature gradient on a length scale (~10 cm), which does not impact the temperature relevant for the atom–surface interaction. In addition, our measurements probe an atom–surface interaction at the level of a single atom, making the ‘temperature’ of the atomic vapour, as an ensemble of moving atoms, irrelevant for our investigation. Atomic vapour and optical pumping For our SR measurements, Cs atoms are first pumped to the 6P 1/2 level, by an 894 nm pump laser. The role of this pump laser is to provide a quasi-thermal velocity distribution of Cs*(6P 1/2 ) atoms at the Cs vapour interface. This was already achieved in previous experiments [23] , [24] . We benefit from collisions, which redistribute the 6P 1/2 excitation to all velocities of both hyperfine components. To avoid any velocity-selective pumping, the pump laser frequency is resonant to the 6P 1/2 hyperfine level, which is not directly probed by the 672-m SR laser (for example, pump reaching the 6P 1/2 ( F =4) level and probe starting from the 6P 1/2 ( F =3) level, or vice versa). The penetration depth of the pumping beam is usually several tens of microns (depending on the exact beam intensity and Cs vapour density). The cell structure and multiple oven design means that the atomic gas is not in equilibrium. Because of collisions, one expects a uniform pressure throughout the cell and a Cs velocity distribution that depends primarily on the local surface temperature. This implies that the Cs density is locally smaller in the hottest areas of the cell, while simultaneously the atomic velocity distribution gets broader. As a result, the SR signal reduces when increasing the temperature of the primary window. This is clearly observed in our measurements ( Fig. 3a ). Optical set-up A distributed bragg reflector laser at 894 nm is used to pump the atoms to the 6P 1/2 intermediate level. The pumping beam is relatively of high power, ~10 mW, with a waist of ~800 μm, and can be sent to the cell on an oblique incidence, practically limited by the geometry of oven 1. An extra on/off amplitude modulation is applied to the pump beam with an acousto-optic modulator, at a frequency of 10 kHz, to improve detection sensitivity. The pump frequency is locked through an auxiliary set-up of SA at 894 nm. The SR probe is an extended cavity laser at 672 nm. The probe beam is slightly smaller, ~500 μm waist, to ensure a complete overlap with the pump, and less powerful, ~50 μW, to avoid saturating the atoms. It is sent to the sapphire window under nearly-normal incidence (on the order of 10 mrad). The laser frequency is scanned by applying a voltage on the piezoelectric element attached to the external grating. The laser is frequency modulated at 1 kHz, with ~5 MHz amplitude. An auxiliary SA experiment and a low finesse Fabry–Perot cavity provide us with frequency markers. An improved method of controlling the frequency scan by beating the probe with a frequency-locked reference laser was also used without any observable improvement in the quality of our SR spectra fits. The reflection of the probe beam is measured with a low-noise photodiode and then demodulated with two cascaded lock-in amplifiers. The atomic signal is typically between four and five orders of magnitude smaller than the reflection from the sapphire/vapour interface. Fitting method C 3 measurements are extracted by fitting experimental spectra to a library of theoretical curves depending on a dimensionless parameter ( A =2 C 3 Γ −1 (2 π / λ ) 3 , with Γ the optical linewidth). Linearity of SR spectroscopy imposes the relative amplitudes and the frequency spacing of the hyperfine components of a given manifold to their theoretical values. The experimental spectrum is compared with a theoretical curve, of a given A , by dilating the frequency axis, to obtain Γ [23] , [24] , [32] , [33] , [34] , [35] . We also allow for an overall offset of the spectrum and adjustment of the global amplitude of the theoretical curve to reflect experimental instabilities. We then change the dimensionless A value and repeat the process until the best fit is identified. This provides a measurement of the C 3 coefficient and the transition linewidth Γ [23] , [24] , [32] , [33] , [34] , [35] . We also allow for a global pressure shift (the same for all hyperfine components). When the above rigid constraints are used, the small differences between the fits and the experimental spectra are probably not entirely of statistical nature. In previous works (see pages 247–248 of ref. 24 ), we have used the frequency spacings and the relative amplitudes between the hyperfine components as free parameters. This slightly improves the fit quality but has negligible effects on the measured values of C 3 and Γ . In the experiment described here, we have restricted the number of free parameters to a minimum. The error bars are conservatively chosen by identifying the values of C 3 and Γ , for which the fit curve falls clearly outside the bounds defined by the noise of the experimental curve [40] . We can also account for a finite Doppler width correction [24] , as the theoretical modelling is essentially developed in the infinite Doppler width approximation. This correction mostly modifies the wings of the SR spectrum. Here, we can safely ignore this correction (attempted for some fittings with no significant changes). This is probably because the width of the hyperfine manifold, which determines the overall lineshape, is much smaller than the Doppler width. How to cite this article: Laliotis, A. et al. Casimir-Polder interactions in the presence of thermally excited surface modes. Nat. Commun. 5:4364 doi: 10.1038/ncomms5364 (2014).